Enantioselective recognition at mesoporous chiral metal surfaces Chirality is widespread in natural systems, and artificial reproduction of chiral recognition is a major scientific challenge, especially owing to various potential applications ranging from catalysis to sensing and separation science. In this context, molecular imprinting is a well-known approach for generating materials with enantioselective properties, and it has been successfully employed using polymers. However, it is particularly difficult to synthesize chiral metal matrices by this method. Here we report the fabrication of a chirally imprinted mesoporous metal, obtained by the electrochemical reduction of platinum salts in the presence of a liquid crystal phase and chiral template molecules. The porous platinum retains a chiral character after removal of the template molecules. A matrix obtained in this way exhibits a large active surface area due to its mesoporosity, and also shows a significant discrimination between two enantiomers, when they are probed using such materials as electrodes. The development of surfaces and materials with chiral features is a major scientific challenge due to the large number of potential applications that can be addressed. Many biological molecules and pharmaceutical compounds are chiral, one enantiomer exhibiting the desired effect while the other one is, in the best case, inactive or can even be toxic. There is thus an increasing demand to either separate enantiomers or to selectively generate them [1] . This results in a continuous growth of the number of methods for asymmetric synthesis [2] , [3] , [4] , [5] , [6] , chiral separation [7] , [8] and selective chiral detection [9] , [10] , [11] , [12] . Although surfaces with chiral characteristics have been successfully obtained by many different approaches, including at the very small scale of metal nanoclusters [13] , [14] , the most popular one is based on molecular imprinting with chiral molecules as templates [10] , [15] , [16] , [17] . This allows designing chiral materials with specific recognition properties, corresponding to the template used [18] , [19] . The approach has been very successfully employed to elaborate molecularly imprinted polymers (MIPs) [20] . However, it sometimes also suffers from disadvantages, such as difficult template removal, poor mass transfer, low binding constants and slow binding kinetics [21] . An alternative way is to generate chirality on metallic surfaces. Chiral metal surfaces have been studied over the past decade and were mainly obtained by one of the following three approaches [22] : (i) cutting a bulk metal along a low symmetry plane, liberating in this way a surface that lacks mirror symmetry [23] , [24] ; (ii) adsorption of chiral molecules at metal surfaces [25] , [26] ; (iii) adsorption of species that play the role of chiral templates on metal surfaces [27] . The limitation of the last two approaches is that the adsorbed chiral molecules can desorb, resulting in weak or no surface chirality [28] . The imprinting approach is expected to lead to intrinsically chiral metal surfaces, retaining their enantioselectivity even after removal of the chiral template. Such surfaces have been successfully produced by electrodeposition of copper oxide films in the presence of chiral tartrate ions. They exhibit moderate enantioselective recognition properties when used for the oxidation of tartrate enantiomers [29] . To date, the synthesis of such intrinsically chiral metal structures by the imprinting approach is still in an early stage of development [30] , [31] . Engineering of chiral Pd, Au, Pt and Ag has been reported [30] , [31] , [32] ; however, the imprinted chirality could not be used for enantioselective recognition after removal of the template. One reason for the low selectivity might be the relatively small surface area, and therefore the small number of imprinted recognition sites, that are available when using flat metal surfaces. Therefore, a promising strategy to improve the amplitude of chiral recognition consists in using porous metals. Mesoporous materials have played an important role in a wide range of applications, such as catalysis [33] , electronic devices [34] , chemical detection [35] and drug delivery [36] . This is because of their attractive features such as high surface area, high stability, well-defined and tunable pore size as well as a predefined organization [37] . Mesoporous metals can greatly improve the accessibility of the metallic framework for guest molecules, and the mesoporous structure can be easily controlled by adapting the lyotropic liquid crystalline phase, which acts as porogen [38] . In the present study, we imprint the structure of chiral molecules at the internal surface of mesoporous platinum. This metal has been chosen since it has a higher structural stability compared with other, much softer metals such as gold. It should therefore retain more efficiently the structure of the template molecule. In contrast to the above-mentioned MIPs, the chiral information is in this case encoded only via the geometry of the cavity and not due to its complementary chemical functionality. This means that, in principle, this approach might be more general and would not need too many adjustments in terms of reagents, when changing the target molecule. Chiral recognition in such porous systems has not yet been demonstrated, even though this would have the twofold advantage of an active surface area that can be two to three orders of magnitude higher compared with flat surfaces, and easy access of the chiral target molecules to the recognition sites. We show that when using such chiral imprinted mesoporous metal surfaces (CIMMS) as electrodes, a very significant discrimination between two enantiomers can be achieved. Engineering mesoporous chiral platinum surfaces In this study, chiral imprinted mesoporous platinum films have been prepared by electrodeposition in the simultaneous presence of a lyotropic liquid crystal phase, which serves as a template to generate the mesopores, and, of the chiral molecule, which acts as the template to obtain chiral cavities in the walls of the mesopores (see Fig. 1 and Methods section for more details of the preparation process). The morphology of the lyotropic liquid crystal chosen for this study is the (H 1 ) phase, leading to an alignment of the final mesopores in a hexagonal lattice [39] . The electrochemical reduction of the metal salt occurs around the lyotropic phase and the chiral molecules. This results in the formation of mesoporous channels with chiral cavities at their inner surface after removal of both types of templates. 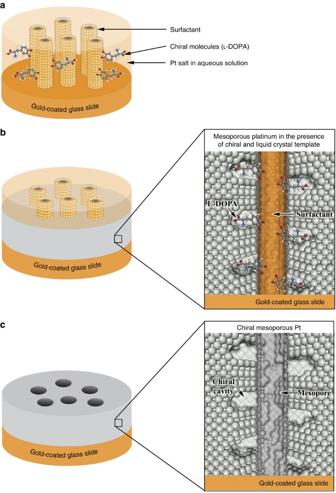Figure 1: Fabrication of chiral-imprinted mesoporous platinum films. (a) Interaction of the liquid crystal phase with the chiral template molecules, (b) Electrodeposition of platinum around the self-assembled structure and (c) Structure after template dissolution. Figure 1: Fabrication of chiral-imprinted mesoporous platinum films. ( a ) Interaction of the liquid crystal phase with the chiral template molecules, ( b ) Electrodeposition of platinum around the self-assembled structure and ( c ) Structure after template dissolution. Full size image L -DOPA (3,4-dihydroxy- L -phenylalanine) has been chosen as the chiral template ( Fig. 2a, I ), since its electroactivity is compatible with the potential window where platinum is subject to neither oxidation nor hydrogen adsorption or evolution. Therefore, when it is used as a probe molecule after the imprinting, its reaction on the platinum electrode can be easily monitored without altering the metal structure. 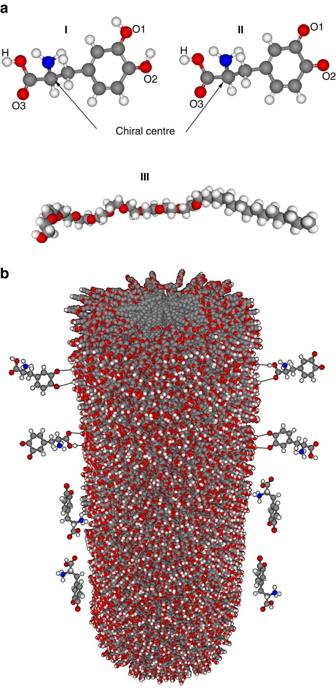Figure 2: Interaction between the chiral molecules and the surfactant phase. (a)L-DOPA (I), the oxidized (quinoic) form ofL-DOPA (II), and the Brij56 surfactant [(C16H33(OCH2CH2)10OH] (III). (b) Schematic view of a column of aggregated Brij56 molecules, present in the lyotropic liquid crystal phase, in interaction with the oxidized DOPA molecules. Figure 2: Interaction between the chiral molecules and the surfactant phase. ( a ) L -DOPA ( I ), the oxidized (quinoic) form of L -DOPA ( II ), and the Brij56 surfactant [(C 16 H 33 (OCH 2 CH 2 ) 10 OH] ( III ). ( b ) Schematic view of a column of aggregated Brij56 molecules, present in the lyotropic liquid crystal phase, in interaction with the oxidized DOPA molecules. Full size image L -DOPA is known to play an important role in pharmaceutics and neurochemistry [40] . DOPA and other catechol compounds have also been employed as reactants to modify inorganic and biological materials [41] , [42] , [43] . Therefore, the transfer of the chiral features from a DOPA enantiomer to the internal pore walls of mesoporous platinum is an interesting choice for this first proof-of-principle study. As the mixture of surfactant and DOPA contains also PtCl 6 2− as platinum precursor, the two hydroxyl groups that are normally located on the aromatic ring of DOPA will be in their quinoic form due to the strong oxidizing character of the platinum salt ( Fig. 2a, II ). DOPA molecules are also pH-sensitive, and the electrodeposition is carried out in a mixture with pH=2, meaning that the protonated form of quinoic DOPA is the molecule present in the mixture. Different interactions of DOPA with the aggregated Brij56 molecules are possible. On the one hand, the two oxygen atoms (indicated as O1 and O2, Fig. 2a ) connected to the ring can be directed towards the hydrophilic surface of the Brij56 columns. On the other hand, the carboxyl group (hydrogen (H) and oxygen (O3) atoms) of the chiral molecule can also interact with the surface of the surfactant phase. Considering the possible establishment of hydrogen bonds between the terminal OH groups of Brij56 and the quinoic part of DOPA as well as the carboxyl group, it is reasonable to assume that the chiral template molecules stay at the outer surface of the surfactant columns and do not penetrate into the hydrophobic core of the columns ( Fig. 2b ). As the platinum salt is dissolved in the aqueous fraction present around the surfactant columns, the metal deposition is expected to occur around the chiral DOPA molecules present at the surface of these template columns, resulting in a transfer of chirality to the walls of the so-generated metallic mesopores. Characterization of mesoporous chiral platinum films To verify the chirality transfer experimentally, platinum-based CIMMS have been generated on gold electrodes. The thickness of the metal film strongly depends on the injected charge density during the electrodeposition. Typically, the thickness of the platinum film varies between 0.3 and 2 μm when charge densities between 2 and 12 C cm −2 are used. Scanning electron microscopy studies show that the thickness of these films is very uniform over the entire area ( Fig. 3a,b ). Transmission electron microscopy reveals a mesoporous structure with pores of about 5 nm diameter ( Fig. 3c ). The active surface area of the porous film is measured by cyclic voltammetry [44] . The voltammograms exhibit the characteristic features of polycrystalline platinum ( Fig. 3d ) with the adsorption and desorption of hydrogen (H a and H d ) and the oxidation and reduction of Pt and PtO n , respectively. The effective active surface area is calculated from the charge associated with the hydrogen adsorption [45] . Compared with a polished flat platinum electrode, the CIMMS show a strong increase in surface area. The calculated surface area is used to estimate a roughness factor, which is defined as the ratio between the active surface area and the geometric surface area of the electrode. Compared with polished platinum, the roughness is increased by a factor of about 80 in the present case. This result confirms that a mesoporous network has been successfully generated. 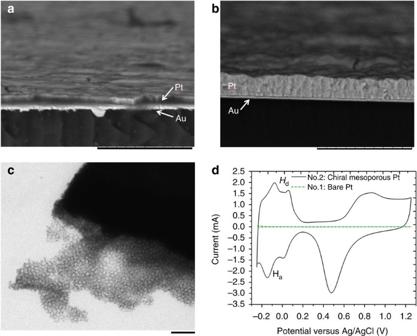Figure 3: Electrode modified with a chiral-imprinted mesoporous platinum film. (a,b) Scanning electron microscopy images of typical cross sections of metal films obtained for injected charge densities of 2 and 12 C cm−2, respectively. Scale bar, 10 μm. (c) Transmission electron microscope image of a chiral mesoporous Pt film. Scale bar, 50 nm. (d) Cyclic voltammograms of flat-polished platinum (No. 1) and a chiral-imprinted mesoporous platinum film obtained by injecting a charge density of 2 C cm−2(No. 2), recorded in 0.5 M H2SO4at 100 mV s−1. Hd(desorption of hydrogen) and Ha(adsorption of hydrogen). Figure 3: Electrode modified with a chiral-imprinted mesoporous platinum film. ( a , b ) Scanning electron microscopy images of typical cross sections of metal films obtained for injected charge densities of 2 and 12 C cm −2 , respectively. Scale bar, 10 μm. ( c ) Transmission electron microscope image of a chiral mesoporous Pt film. Scale bar, 50 nm. ( d ) Cyclic voltammograms of flat-polished platinum (No. 1) and a chiral-imprinted mesoporous platinum film obtained by injecting a charge density of 2 C cm −2 (No. 2), recorded in 0.5 M H 2 SO 4 at 100 mV s −1 . H d (desorption of hydrogen) and H a (adsorption of hydrogen). Full size image Electrochemical enantioselectivity To illustrate the enantioselective properties of such CIMMS, the electrodes were studied by differential pulse voltammetry (DPV). As shown in Fig. 3d , different electrochemical processes, including hydrogen sorption and the oxidation of platinum, can occur during a scan of the potential. To avoid interference of these reactions with the enantioselective recognition, the electrochemical activity of the probe molecule should be located in a potential range where no such competing faradaic processes occur (typically in the range between 0.2 and 0.7 V). It is therefore important to note that DOPA undergoes electro-oxidation in a potential window between 0.35 and 0.60 V. From an electrochemical point of view, the behaviour of L -DOPA and D -DOPA on non-imprinted flat platinum electrodes is, as expected, identical ( Fig. 4a ). In addition, the DPV responses of the two enantiomers are also identical on non-imprinted mesoporous platinum ( Supplementary Fig. 1 ). From these observations it is clear that the two enantiomers, as expected, cannot be discriminated on both non-imprinted flat and mesoporous electrodes. However, the current density of DOPA electro-oxidation on non-imprinted mesoporous platinum is strongly increased compared with a flat polished platinum electrode (shown in Supplementary Fig. 1b ). 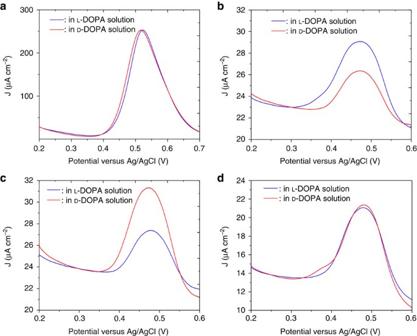Figure 4: Characterization of the enantioselectivity by differential pulse voltammetry. DPV in 4 mML-DOPA (blue) andD-DOPA (red) using 50 mM HCl as supporting electrolyte with (a) a flat platinum electrode, (b) a chiral mesoporous platinum electrode imprinted withL-DOPA using aL-DOPA/ PtCl62−ratio of 1/25, (c) a chiral mesoporous platinum electrode imprinted withD-DOPA using aD-DOPA/PtCl62−ratio of 1/25, (d) chiral mesoporous platinum electrodes initially imprinted withL-DOPA, but measured after deliberately destroying the chiral information by scanning the potential between -0.2 V and +1.25 V in 0.5 M H2SO4. Figure 4: Characterization of the enantioselectivity by differential pulse voltammetry. DPV in 4 mM L -DOPA (blue) and D -DOPA (red) using 50 mM HCl as supporting electrolyte with ( a ) a flat platinum electrode, ( b ) a chiral mesoporous platinum electrode imprinted with L -DOPA using a L -DOPA/ PtCl 6 2− ratio of 1/25, ( c ) a chiral mesoporous platinum electrode imprinted with D -DOPA using a D -DOPA/PtCl 6 2− ratio of 1/25, ( d ) chiral mesoporous platinum electrodes initially imprinted with L -DOPA, but measured after deliberately destroying the chiral information by scanning the potential between -0.2 V and +1.25 V in 0.5 M H 2 SO 4 . Full size image In strong contrast to this, the chiral imprinted mesoporous platinum shows significant differences in the electro-oxidation current densities between L -DOPA and D -DOPA. We found that chiral mesoporous platinum electrodes imprinted by L -DOPA are much more active with respect to the electrooxidation of L -DOPA compared with that of D -DOPA ( Fig. 4b ). In contrast, those electrodes imprinted in control experiments with D -DOPA are more active for D -DOPA oxidation ( Fig. 4c ). This difference in activity can be attributed to the chiral ‘footprints’ that have been generated in the pore walls during the imprinting process, thus facilitating the oxidation of the DOPA molecules that have the right configuration. To quantify the enantioselectivity in both cases 4b and 4c, one needs to compare the relative current changes. If these values are calculated by taking the absolute current differences and dividing them by the peak current of the imprinted species with respect to the baseline, ~0.4 is obtained for both sets of experiments. This means that there is a 40% decrease of current when comparing the signal of the imprinted versus non-imprinted species. Small variations between two sets of experiments can be attributed to the fact that different parameters, like for example temperature, can have an impact on the efficiency of the imprinting process. To exclude that the observed enantioselectivity is generated by a layer of DOPA molecules remaining inside the pores, even after extensive washing of the electrodes after the imprinting process, we carried out a series of control experiments. Indeed DOPA is known to adsorb on platinum [46] , [47] , and this could eventually lead to supramolecular diastereomeric interactions with DOPA molecules in solution, leading in fine to chiral discrimination. Such a mechanism could be excluded as shown in Supplementary Figs 2–7 ). To verify that no other artifacts, such as a change in active surface area, lead to these observations, we carried out another control experiment. As stated above, and also illustrated in Fig. 3d , for potentials more positive than 0.6 V the platinum surface starts to become oxidized. When performing such an oxidation, followed by the back-reduction of the formed platinum oxide, the platinum atoms at the inner surface of the pore walls, that initially encode the chiral information, will reorganize. This should erase the chiral surface imprints. To verify this effect, the electrooxidation of L -DOPA and D -DOPA was reinvestigated once the electrodes had been oxidized and reduced during a full potential cycle in sulfuric acid from −0.25 to 1.25 V and back. In this case, no selectivity between the two enantiomers is found ( Fig. 4d ), confirming that oxidation of the chiral-imprinted mesoporous material destroyed its chirality. The active surface areas of all chiral electrodes are obtained by cyclic voltammetry experiments ( Supplementary Fig. 8 ), subsequent to the chiral recognition DPV experiment. This allows the renormalization of the current densities to compare all electrodes with each other, and Fig. 4d confirms that the electrodeposition process itself is very reproducible. The enantioselective recognition properties should depend on the amount of imprinted recognition sites. We therefore carried out several experiments with varying amounts of DOPA in the electroplating mixture. The enantioselectivity, calculated from the electro-oxidation current density ratio of L -DOPA to D-DOPA (J L -dopa /J D -dopa ), significantly rises when the content of chiral template is increased. For instance, the current density ratio of L -DOPA to D -DOPA increases from 1.2 to 2.4 for a chiral-imprinted mesoporous electrode obtained using L -DOPA/PtCl 6 2− molar ratios of 1/50 and 1/17, respectively. The reason for this increase in enantioselectivity relates to the fact that the increase of the chiral template content is directly influencing the number of created chiral cavities in the mesoporous structure. In contrast, for even higher amounts of chiral template (molar ratio of L-DOPA/PtCl 6 2− >1/12), the efficiency of the enantioselective recognition starts to decrease. This is most likely due to the fact that a large concentration of chiral template destabilizes the lyotropic liquid crystal phase of the surfactant used as mesopore directing agent. An indication for this is the observation that in the presence of large concentrations of DOPA template, the final metal layer is much more brittle and tends to detach from the electrode surface. To illustrate the beneficial effect of mesoporosity on the enantioselectivity, the chiral recognition of the two enantiomers of L - and D -DOPA was also investigated on chiral imprinted non-mesoporous platinum deposits. In this case, the electrode was simply prepared by an electrochemical reduction of the platinum salt in the presence of the chiral molecules ( L -DOPA/Pt=1/25), but without surfactant. Interestingly, only a slight difference in the electro-oxidation current is observed between the two enantiomers ( Supplementary Fig. 9 ). This makes it clear that the mesoporous structure is a crucial feature for the enantioselectivity because almost no chiral cavities seem to be generated in the absence of surfactant. This is consistent with the view that the chiral cavities in the walls of the mesopores are generated due to the interaction between DOPA and the surfactant molecules, trapping DOPA on the surface of the pillars of the lyotropic liquid crystal phase. The chiral templates seem to remain in this position during the reduction of the platinum salt, whereas in the absence of surfactant only a few chiral recognition sites are imprinted on the outermost surface of the platinum layer. As a result, a significant discrimination between the two enantiomers of DOPA is observed for the mesoporous structure, whereas the non-mesoporous platinum deposit shows only a very modest selectivity. It was also found that the mechanical stability of chiral imprinted non-mesoporous platinum films is low, they are easily destroyed during oxidation by cyclic voltammetry in sulfuric acid, whereas the films of chiral mesoporous platinum are stable, even when the electrode is oxidized and reduced several times. Enantioselective adsorption It has been reported [24] , [26] that enantioselective properties at metal surfaces can be successfully generated by introducing defects, for example, steps, kinks and vacancies on the metal, resulting in slightly different adsorption energies for the two enantiomers at such surfaces. It is therefore reasonable to assume that in the case of the imprinting approach it should also be possible to generate sites with different adsorption enthalpies for the two enantiomers. Macroscopically, this should lead to a difference in partition coefficient between the outer solution phase and the inside of the porous structure when comparing the two enantiomers. To confirm this hypothesis, adsorption experiments were performed by exposing chiral mesoporous platinum films to racemic mixtures of L -DOPA and D -DOPA and monitoring the composition of the supernatant solution by HPLC with a chiral stationnary phase. In Table 1 , the D / L DOPA separation factors ( α D / L ) were calculated as the quotient of the ratios of D -DOPA to L -DOPA concentrations in the solution, after and before being in contact with the platinum films for a certain time (1, 3 and 5 h). The α D / L of a non-imprinted mesoporous platinum film (NIM-Pt 4C cm −2 ) is, as expected, close to one, within experimental errors, even after an adsorption time of 5 h (Entry 1), implying no enantioselective adsorption on such materials. In contrast, the chiral mesoporous platinum films obtained with L -DOPA as chiral template (CIM-Pt-L 4C cm −2 ) show a significant increase in enantioselectivity, especially after longer exposure times (Entry 2). It is noteworthy that this characteristic time is much longer than the duration of the electrochemical experiments. This may be explained by the fact that dry platinum films were used for the adsorption experiments, while the electrochemical experiments were carried out with already wet electrodes. The wetting and the diffusion of DOPA into the mesoporous channels takes more time in the case of an initially dry electrode. Table 1 Enantioselective adsorption of a racemic DOPA solution on chiral mesoporous platinum films. Full size table The α D / L values were compared for different experimental conditions. When increasing the thickness of the platinum film by using a higher injected charge density during the electrodeposition, the enantioselective adsorption does not change very much at room temperature (22 °C) (Entries 2 and 3). However, the enantioselective adsorption is significantly increased at low temperature (Entry 4). The α D / L at 22 and 2 °C of chiral mesoporous platinum, imprinted by L -DOPA for an injected charge density of 8 C cm −2 , is 1.32 and 1.52, respectively. This indicates that L -DOPA is preferentially adsorbed in the metal matrix, leaving an excess of D -DOPA in the supernatant phase. The opposite effect is observed for chiral platinum films that have been imprinted with D -DOPA. The α D / L becomes smaller than 1, suggesting that the adsorption of D -DOPA is favoured in these materials (Entries 5 and 6). Interestingly, an increase in thickness leads to a more pronounced change in enantioselectivity when measured at low temperatures (Entries 5 and 6), compared with what is observed at higher temperatures (Entry 2 and 3). Although the difference is not very large, this is in agreement with an energetic stabilization of the preferred adsorption state in such imprinted materials [48] , [49] . The obtained results indicate that applying the general philosophy of molecular imprinting to organized porous metals, having high surface areas, results in CIMMS that show a very significant selectivity for one or the other enantiomer. Control experiments could exclude that this selectivity is due to the presence of chiral molecules left over in the cavities after imprinting. The observed enantioselectivity strongly depends on several parameters, like the thickness of the imprinted metal layer, the type and amount of chiral template present during the imprinting, as well as the temperature. Playing with these parameters allows the rational design of enantioselective surfaces, but, depending on the surface mobility of the metal atoms, not all metals might be equally appropriate for maintaining the chiral information. In conclusion, our results demonstrate that mesoporous platinum with a pronounced chiral character has been successfully obtained by electrodeposition of platinum in the simultaneous presence of a surfactant, forming a lyotropic crystal phase and a chiral template molecule. Because of interactions between the surfactant and the chiral template, it has been possible to generate chiral footprints in the mesopores, allowing the discrimination between two enantiomers in electrochemical and adsorption experiments. The effect of this chirality transfer from a molecular species to a metal phase is amplified by the high active surface area of the mesoporous matrix. This first example of a chiral imprinted metal, which retains its chirality even after removal of the template, is complementary to the family of molecular imprinted polymers, and it opens up interesting perspectives for the development of new materials for a wide range of applications from chiral synthesis and enantioselective sensing to chiral separation and purification. Chemicals Hexachloroplatinic acid hydrate (H 2 PtCl 6 . xH 2 O), polyoxyethylene (10) cetyl ether (Brij 56), 3,4-dihydroxy- D -phenylalanine ( D -DOPA), 3,4-dihydroxy- L -phenylalanine ( L -DOPA) and the racemic mixture of 3,4-dihydroxy- DL -phenylalanine ( DL -DOPA) were purchased from Sigma-Aldrich (Missouri, USA). 1 M hydrochloric acid (HCl) was purchased from J.T. Baker (Deventer, Holland). All chemicals were used without further purification. All solutions were prepared with milliQ water. Synthesis of chiral-imprinted mesoporous platinum electrodes Liquid crystal plating mixtures were prepared as a quaternary system composed of 42 wt% of nonionic surfactant (Brij 56), 29 wt% of chloroplatinic acid, 29 wt% of DI water and the desired amount of L -DOPA or D -DOPA. Electrochemical reduction of platinum salts in the presence of surfactant and DOPA enantiomer was carried out at −0.1 V on gold-coated glass slides (0.25 cm 2 ). After the electrodeposition process, the prepared samples were rinsed for several hours with a large amount of water to remove the surfactant and the chiral template. To ensure the complete removal of the chiral template during the washing, all electrodes were checked by differential pulse voltammetry (DPV) in 50 mM HCl for the electrochemical signal of eventually remaining DOPA. Only completely DOPA-free electrodes were used for the subsequent experiments. For non-imprinted mesoporous platinum, the plating mixture was a ternary system composed of 42 wt% of Briji 56, 29 wt% of chloroplatinic acid and 29 wt% of DI water. For generating chiral-imprinted non-mesoporous platinum electrodes, the electrodes were prepared by electrodeposition at −0.1 V in an aqueous mixture of 60 mM chloroplatinic acid and L -DOPA ( L -DOPA/Pt=1/25) without adding surfactant. Characterization and chiral recognition studies SEM and TEM experiments were carried out on a Hitachi TM-1000 tabletop microscope and a JEOL JEM-2010 TEM, respectively. For TEM measurements, chiral-imprinted mesoporous platinum films on Au-coated glass slides were exposed to an aqueous solution of 4 wt% KI and 1 wt% I 2 for 20 min to dissolve the underlying Au layer. The Pt film could then be easily removed from the electrode and floated on the water surface after slow immersion of the samples into DI water. The freestanding films were then transferred onto TEM grids. All electrochemical experiments were performed with a μ-Autolab Type III using Ag/AgCl (sat. KCl), a Pt mesh and the prepared mesoporous electrodes as reference, counter and working electrodes, respectively. The chiral recognition studies were based on two independent techniques. The first one is differential pulse voltammetry (DPV). The parameters of the DPV used here were a pulse modulation of +50 mV in amplitude, a pulse duration of 50 ms and an interval time of 0.1 s. The second technique is based on adsorption experiments, exposing a 100 μM racemic mixture of DL -DOPA to the chiral-imprinted mesoporous platinum layers (0.25 cm 2 ), obtained by injecting various charge densities during the electroplating. After a certain time, the supernatant solution was collected and analyzed by HPLC. HPLC was performed on a Merck L-6200A instrument with detection at 230 nm using a UV detector (L-4000A Model). The HPLC analytical assays were carried out on a 150 mm × 3 mm ID CHIRALPAK ZWIX (+) column (Chiral Technologies Europe). All analyses were performed at a flow rate of 0.5 ml min −1 , using as mobile phase a mixture of 50/50 (v/v) methanol/acetonitrile and 50 mM formic acid as well as 25 mM diethylamine. Before analysis of the samples by HPLC, the remaining supernatant solution was evaporated to remove all solvent, and redissolved in the mobile phase. How to cite this article: Wattanakit, C. et al . Enantioselective recognition at mesoporous chiral metal surfaces. Nat. Commun. 5:3325 doi: 10.1038/ncomms4325 (2014).